Large microwave generation from current-driven magnetic vortex oscillators in magnetic tunnel junctions Spin-polarized current can excite the magnetization of a ferromagnet through the transfer of spin angular momentum to the local spin system. This pure spin-related transport phenomenon leads to alluring possibilities for the achievement of a nanometer scale, complementary metal oxide semiconductor-compatible, tunable microwave generator that operates at low bias for future wireless communication applications. Microwave emission generated by the persistent motion of magnetic vortices induced by a spin-transfer effect seems to be a unique manner to reach appropriate spectral linewidth. However, in metallic systems, in which such vortex oscillations have been observed, the resulting microwave power is much too small. In this study, we present experimental evidence of spin-transfer-induced vortex precession in MgO-based magnetic tunnel junctions, with an emitted power that is at least one order of magnitude stronger and with similar spectral quality. More importantly and in contrast to other spin-transfer excitations, the thorough comparison between experimental results and analytical predictions provides a clear textbook illustration of the mechanism of spin-transfer-induced vortex precession. The spin-transfer torque due to the interaction between a spin-polarized current and magnetization [1] , [2] has led in the last decade to the emergence of a number of interesting novel effects such as current-induced magnetization reversal [3] , [4] or self-sustained magnetization oscillations [5] , [6] . The observation of spin-transfer-induced magnetization precession brings some promising possibilities for designing a new type of nanoscale microwave oscillators, called spin-transfer nano-oscillators (STNOs), capable of competing with currently used millimeter-scale microwave synthesizers in terms of characteristics of the emission. One of the tantalizing qualities of STNOs is that they are tunable over a wide frequency range by varying the applied direct current (DC) or magnetic field. In most experiments performed up to now [5] , [6] , current-induced excitations were quasi-uniform precessions in purely metallic structures, which generate a microwave power that is too small for the majority of applications. Various solutions have been recently proposed, for example, synchronizing an assembly of STNOs [7] , [8] , [9] , [10] , [11] or using MgO-based magnetic tunnel junctions (MTJs) [12] , [13] , which deliver much larger power because of an increased magnetoresistance (MR) [14] , [15] , [16] . However, the spectral linewidths of MgO MTJs are still too large (≈100 MHz) for standard excitations of the free layer in MTJs because of the chaotic behaviour induced by the spin-transfer torque and/or high non-linearity [17] . An alternative approach using the current-driven motion of a magnetic vortex as a source of microwave power has been recently studied in metallic nanopillars [18] . A very interesting mode is the circular motion of the vortex core around its equilibrium position [19] . This low-energy mode gives rise to very small linewidths (<1 MHz) in the sub-GHz range, but generates only a very small integrated power in all metallic devices (≈0.01 nW). In this paper, we show that large microwave powers and narrow linewidths can be obtained simultaneously by spin-transfer-induced vortex motion in MgO MTJs. Spin-transfer vortex oscillator The studied devices are circular shaped nanopillars with a diameter ( d )=170 nm patterned from a magnetic stack: synthetic antiferromagnet (SAF)/MgO 1.075 nm/NiFe 15 nm/capping. For the chosen parameters of NiFe thickness and dot diameter, we have checked that the most favourable configuration is a single vortex state (see Methods and Supplementary Fig. 1 ). In these nano-MTJs, vortex dynamics are converted into a microwave signal because of the large magnetoresistive ratio of the tunnel MR (TMR) effect. This enables us to detect not only large sustained vortex oscillation induced by spin transfer but also small signals associated with the ferromagnetic resonance of the thermally excited vortex. Such resonant motion is efficient enough to produce competitive passive microwave elements such as high-gain resonators [20] , [21] . In Fig. 1a , we display some microwave emission spectra recorded with H perp =+5.1 kOe at several positive current values. For all I dc values, a single peak is observed in the sub-GHz frequency range that is characteristic of the coherent gyrotropic motion of the magnetic vortex core that is induced by spin-transfer torque [18] . Emission frequency increases with I dc (≈80 MHz mA −1 ), together with a large increase in the peak power spectral density. The best results have been obtained at large currents ( I dc =3.2 mA) but still below the threshold above which MTJ is damaged. At this value, the peak linewidth is only 1.1 MHz and the integrated power is about 5 nW. This is to our knowledge the highest emitted power for STNOs exhibiting similar linewidths. It therefore shows the interest to use the motion of a vortex as a microwave source, as we benefit from the advantages of both the coherency of the vortex gyrotropic motion and the large magnetoresistive signal provided by an MTJ. 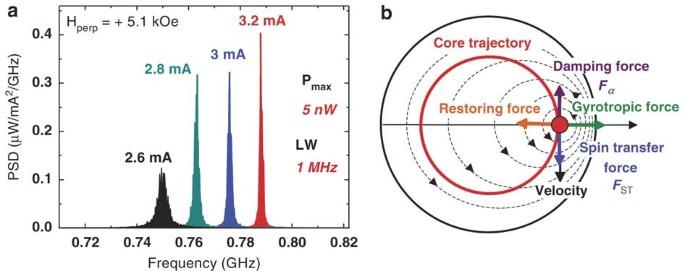Figure 1: Large microwave emission spectra associated with vortex oscillations. (a) Power spectral densities (PSD) normalized by/dc2, obtained forIdc=2.6, 2.8, 3 and 3.2 mA withHperp=5.1 kOe. (b) Schematic of the different forces having an effect on the vortex core. Figure 1: Large microwave emission spectra associated with vortex oscillations. ( a ) Power spectral densities (PSD) normalized by/ dc 2 , obtained for I dc =2.6, 2.8, 3 and 3.2 mA with H perp =5.1 kOe. ( b ) Schematic of the different forces having an effect on the vortex core. Full size image Conditions for sustained vortex oscillations With regard to spin-transfer-induced excitations of quasi-uniform magnetization configurations, little comparison has been made between experimental results and theoretical predictions. This is mainly because of difficulties in accurately taking into account the presence of multi-mode excitations, the different sources of spin-transfer torques and the roles of the Oersted field or temperature [22] . An important aspect of our work is that we provide a definite comparison and an excellent agreement between experimental data, micromagnetic simulations and analytic predictions. As a matter of fact, we show that our experiments can be interpreted in the frame of the most recent theoretical descriptions of the spin-transfer-induced vortex gyrotropic motion using a modified Thiele equation [23] , [24] , [25] . The starting point is the Thiele equation including the spin-transfer torque: where G =−2π pLM s / γ e z is the gyrovector, with p the core polarity, L the thickness of the NiFe layer, M s the saturation magnetization, γ the gyromagnetic ratio and e z the unit vector along the normal direction. W( X ) is the potential of the off-centre vortex, where X is the core position, and D̂ is the damping dyadic. In Fig. 1b , we depict the four forces responsible for the rotational motion of the vortex core around its equilibrium position. In equation (1), the first two terms, corresponding, respectively, to the gyrotropic force and the restoring force, are radial with respect to the vortex trajectory, and their balance sets the frequency of motion. The last two terms, corresponding, respectively, to viscous damping (later denoted as F α ) and the spin-transfer force, F ST , are tangent to the trajectory, and their compensation sets the amplitude of the orbit. It is to be noted that we introduce only the Slonczewski term for the spin-transfer torque. The field-like term, being equivalent to an additional applied magnetic field directed along the polarizer, has been neglected, as its amplitude is small compared with the applied H perp [26] . In the case of a fixed and uniform polarizer, we derive an expression for the spin-transfer force F ST given by [23] where σ is the spin-transfer efficiency (equal to h̄P spin /2| e | LM s , with P spin being the spin polarization of the current), L is the thickness of the dot, J is the current density (defined as positive for electrons flowing from the NiFe layer to SAF layers), a is the orbit radius and e χ is the unit vector tangential to the orbit of the core. The spin-transfer force F ST is proportional to p z , the out-of-plane component of the polarizer ( p z =cos θ , if θ is the angle between the magnetization and the out-of-plane direction). The expression of the damping force F α is where α is the damping constant, is a damping parameter, Ê is a unit tensor, and ω is the rotational speed. The sign of the core velocity, and consequently the sign of F α , depends on the polarity p of the vortex core, which is: p =1 when the core is pointing upwards and p =−1 when it is pointing down. The condition for the sustained gyration of the vortex core is that the spin-transfer force should counterbalance the damping. It follows from the respective signs of equations (2, 3) that spin-transfer-induced vortex oscillation should be observed only if the vortex core and the polarizer are pointing in the same direction when the current is positive, and if they point in opposite directions when the current is negative, compared with metallic devices. Our MgO-based nano-oscillators are model systems to test these theoretical predictions. The reasons are twofold. First, the SAF structure of the polarizer provides a uniform and fixed spin polarization. Second, the current amplitude is small enough to avoid tilting of the polarizer by the Oersted field or induced dynamics in the SAF. Overview of the vortex dynamics We plot in Fig. 2 the integrated microwave power for I dc =3.2 mA (top panel) and the frequency for two values of I dc (bottom panel) as a function of the out-of-plane magnetic field H perp . The field is swept from −8.1 to 8.1 kOe and the out-of-plane component of the polarization p z is expected to be proportional to | H perp |. 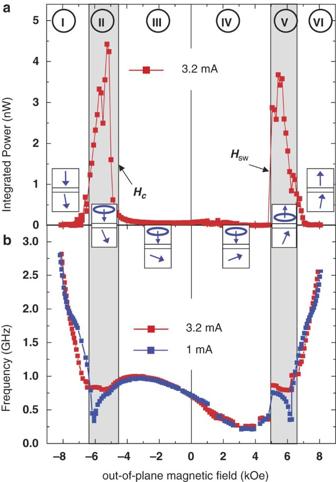Figure 2: Power and frequency dependence on the magnetic field. (a) Integrated power as a function of the out-of-plane magnetic field. The field is swept from negative to positive values.Hcis the critical field at which microwave oscillations occur forIdc=3.2 mA,HSWis the field at which the vortex core reverses. (b) Frequency as a function of the out-of-plane magnetic field. Blue dots:Idc=1 mA, red dots:Idc=3.2 mA. Figure 2: Power and frequency dependence on the magnetic field. ( a ) Integrated power as a function of the out-of-plane magnetic field. The field is swept from negative to positive values. H c is the critical field at which microwave oscillations occur for I dc =3.2 mA, H SW is the field at which the vortex core reverses. ( b ) Frequency as a function of the out-of-plane magnetic field. Blue dots: I dc =1 mA, red dots: I dc =3.2 mA. Full size image Considering first the variation of the integrated power as a function of the out-of-plane field in the top panel of Fig. 2 , we can identify the following successive zones. In zone I, for H perp <−7.5 kOe, the absolute field value is large enough to induce a uniform magnetic configuration (no vortex) and the power is negligibly small. In zone II, a vortex comes out and, as the vortex core polarity and the out-of-plane component of the polarization H z are both negative, a vortex gyration is induced and a large microwave power is emitted (about 5 nW at I dc =3.2 mA). When | H perp | becomes smaller than H c ≈4.5 kOe (zone III), the out-of-plane polarization p z is too small to excite large gyration and the power is negligible at the scale of the figure. In zone IV, not only is | p z | too small for H perp < H c but, with the inversion of H perp , the vortex core polarity and the polarizer have opposite signs. The condition for vortex gyration is not satisfied and, even for H perp > H c , the power remains very small (max. 270 pW at I dc =3.2 mA). In zone V, which begins at H SW =5 kOe, the switching of the vortex core aligns p and p z , which induces gyration and large microwave power. Finally, in zone VI, for H perp >6.5 kOe, as in zone I, there is no vortex present and the power is negligible. The variation of frequency as a function of the field in the bottom panel of Fig. 2 fits with the variation of the power discussed above. For | H perp |>7.5 kOe (zones I and VI), the magnetic field is strong enough to saturate the magnetization of the NiFe layer for all I dc values, and a spatially uniform configuration with the magnetization pointing out-of-plane is stabilized. The frequency of excitation increases linearly with the field, independently of the current I dc , as expected from the ferromagnetic resonance Kittel formula for small-amplitude uniform precession. In this large-field region, the slope is close to the expected value of 2.8 GHz kOe −1 and the intercept with the zero-frequency axis occurs at 7.7 kOe, which corresponds to 4π M s NiFeM =9 kOe after taking into account demagnetizing factors. For | H perp | between 6.5 and 7.5 kOe, one clearly observes in Fig. 2a , a slight deviation from the Kittel mode, reflecting the onset of a weak inhomogeneity that is suppressed when I dc increases. Such behaviour is well reproduced by the micromagnetic simulations of the frequency versus the out-of-plane magnetic field presented in Fig. 3 , in which a small tilt (1°) of H perp from the normal direction is introduced. In both zone I and VI, as mentioned before, very low power emission is measured in agreement with that which is generally observed for a uniform magnetization oscillation of the free layer. 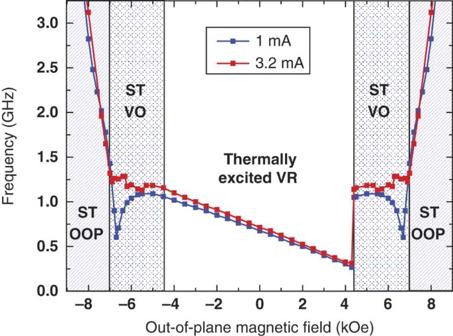Figure 3: Micromagnetic simulations: frequency versus the out-of-plane magnetic field forIdc=1 and 3.2 mA. Different regimes are identified, namely, spin transfer-induced out-of-plane uniform precession (ST-OOP), spin transfer vortex oscillation (ST-VO) and thermally excited vortex resonance (VR). The field is swept from negative to positive values. Figure 3: Micromagnetic simulations: frequency versus the out-of-plane magnetic field for I dc =1 and 3.2 mA. Different regimes are identified, namely, spin transfer-induced out-of-plane uniform precession (ST-OOP), spin transfer vortex oscillation (ST-VO) and thermally excited vortex resonance (VR). The field is swept from negative to positive values. Full size image The transition between uniform magnetization and vortex configuration (zone II) occurs at H perp =−6.1 kOe (the inverse transition (zone V) occurs at H perp =6.1 kOe). It is characterized by a dip in frequency, as can be observed from the curve at I dc =1 mA in Fig. 2 . This dip is well reproduced by the micromagnetic simulation results shown in Fig. 3 , and is related to a modification of the shape of the vortex core that results in a softening of the mode. In this field range of large emission, the simulation for I dc =3.2 mA is in good agreement with the experimental results. We find that the combined action of the spin-transfer torque and the Oersted field strongly modifies the evolution of the frequency and stabilizes the vortex configuration to larger H perp (see Supplementary Fig. 2 for the observation of the gradual disappearance of the frequency dip as the current is increased). In the experiment and simulation, we see that several large-amplitude non-uniform oscillating modes are successively excited when changing the field. We note that such a sequential transition of modes is not detectable by measuring the resistance-field dependence of the device. Below the critical field | H c |, only a thermally excited vortex motion associated with a very small power is observed and, in consequence, the two frequency curves at different I dc values are superimposed (see Fig. 2b ). While increasing H perp from −4.5 to + 4.9 kOe (that is, zones III and IV), after a small increase in frequency, the general trend is a decrease in the gyrotropic frequency (see Fig. 2 , top panel), as already observed for alternating current field-induced vortex resonance in a study conducted by De Loubens et al . (see equation 2 in Ref. 27 ), and is due to field-dependent vortex stiffness. The deviation from the expected linear behaviour of the frequency versus field behaviour is attributed to a deformation of the energy landscape by grains. For H SW =+5 kOe, a large jump in frequency occurs because of the reversal of the vortex core polarity. After switching, it becomes aligned to the applied field and to the polarizer, as in the case of large negative fields (zone I). The reversal of the core polarity, associated with the abrupt change in frequency and the recovery of the oscillation, is well reproduced by simulation (see Fig. 3 ). It is worth emphasizing that a symmetrical behaviour is obtained when saturating first in a large positive H perp and then decreasing the field towards negative values. As already mentioned, for negative currents, the condition to obtain large oscillations is that the vortex core polarity and the out-of-plane component have opposite signs. The measurement of the integrated microwave power for I dc =−5 mA as a function of H perp , swept from −8.1 to 8.1 kOe, is presented in Fig. 4 . A large microwave power is detected in a very narrow field window between H c =3.7 kOe and H SW =4.3 kOe. We notice that H SW is reduced because the vortex motion with a finite velocity, induced at negative currents, promotes the core switching at lower magnetic field [28] . This implies that we have to increase the absolute value of the injected current to decrease H c and fulfil the condition H c < H SW . The counterpart of this additional experimental verification of the model is that we must have used a DC that damages the junction quality and leads to a decrease in the MR ratio, and therefore we got a smaller microwave output power as compared with positive currents. 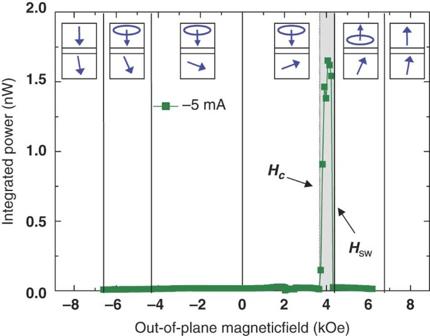Figure 4: Integrated power as a function of the out-of-plane magnetic field for a negative current. The field is swept from negative to positive values.Hcis the critical field at which microwave oscillation occurs forIdc=−5 mA,HSWis the field at which the vortex core reverses. Figure 4: Integrated power as a function of the out-of-plane magnetic field for a negative current. The field is swept from negative to positive values. H c is the critical field at which microwave oscillation occurs for I dc =−5 mA, H SW is the field at which the vortex core reverses. Full size image Quantitative comparison with the model To extract quantitative information about the spin torque force, an expression of the critical current density J c for the onset of sustained vortex oscillations can be obtained by equalizing equations (2,3). By this calculation, we predict that the ratio f / J c between the frequency and the critical current density should be proportional to the out-of-plane polarization p z : In our magnetic system, the spin polarization comes from the CoFeB layer of the SAF. Thus, the evolution of p z with the out-of-plane magnetic field can be expressed by p z = H perp /4π M s SAF . The ratio f / J c is expected to vary linearly with H perp . In Fig. 5 , we plot the experimental values of f / J c versus the out-of-plane magnetic field for increasing (blue squares) and decreasing (red squares) values of the field. The expected linear variation of f / J c with H perp is clearly confirmed by the experiments. In Fig. 5 , we also plot, in solid lines, the result of an analytical calculation using equation (4), taking 4π M s NiFe =9.0 kOe, 4π M s SAF =10.3 kOe, α=0.01, η =1.48 and P spin =0.53. We emphasize that this value of P spin is consistent with the MR ratios in conventional CoFeB/MgO/CoFeB MTJs in which P spin =0.5–0.6 for the CoFeB/MgO interface using the simple Julliere's model. The excellent agreement between the experimental results and the theoretical predictions on the whole field range reveals that not only a qualitative but also a quantitative understanding of the spin-transfer vortex dynamics has been achieved. 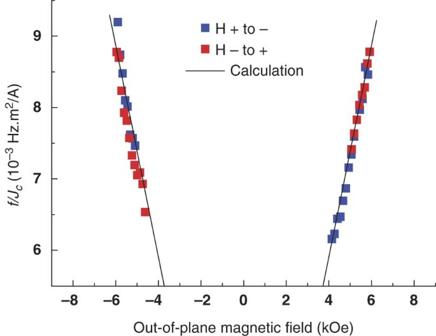Figure 5: The ratio of frequency to critical current density as a function of the out-of-plane magnetic field for both sweep directions. Red symbols: negative to positive, blue symbols: positive to negative. Black lines correspond to the calculations using equation (4). Figure 5: The ratio of frequency to critical current density as a function of the out-of-plane magnetic field for both sweep directions. Red symbols: negative to positive, blue symbols: positive to negative. Black lines correspond to the calculations using equation (4). Full size image Role of grains on vortex dynamics The location of the vortex core inside the nanodot can also strongly influence its dynamical properties. This core position can be controlled by the application of an in-plane magnetic field H in that forces the vortex to move perpendicularly to the field [29] . In addition, it provides a tool to investigate the role of material grains on the motion of vortices and also potentially increase the accessible frequencies. In Fig. 6a , we display the measurement of the gyrotropic mode frequency as a function of H in . We observe an oscillating behaviour of the frequency while the magnetic vortex travels from the centre of the dot where it is nucleated to the edge of the disk where it is annihilated. Such large frequency variations are due to the modification of the magnetization and/or the local anisotropies at the grain boundaries that changes the pinning potential [30] , [31] , [32] . From this measurement, the number of material grains in the nanodot can be evaluated. We deduce a grain size of about 40 nm in agreement with the AFM measurements shown in Fig. 6b . Interestingly, we find that when the resonance frequency is low (high), thermally induced vortex fluctuations are enhanced (reduced), as shown in Fig. 6a . This is because for a lower (larger) stiffness of the potential well probed by the vortex core, the amplitude of the core motion is larger (smaller) at a given excitation level. 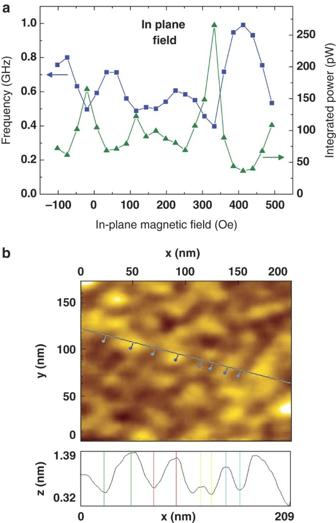Figure 6: Evolution of frequency and power with in-plane magnetic field. (a) Left axis (blue squares): frequency, right axis (green triangles): integrated power as a function of the in-plane magnetic field. (b) Atomic Force Microscopy topography image of the NiFe layer. Bottom: scan of thickness as a function of location. Figure 6: Evolution of frequency and power with in-plane magnetic field. ( a ) Left axis (blue squares): frequency, right axis (green triangles): integrated power as a function of the in-plane magnetic field. ( b ) Atomic Force Microscopy topography image of the NiFe layer. Bottom: scan of thickness as a function of location. Full size image Future directions The perspective opened by our results is very promising. From an applications point of view, we have shown that the current-induced excitation of a vortex in a low-resistivity MTJ, having an MR ratio of only 10%, can lead to microwave emission characterized by both a large power (5 nW) and a narrow linewidth (1 MHz). Furthermore, the excellent agreement between our experiments and theory signifies that our results are a textbook example of the physics of current-induced vortex gyrations. Interestingly, our work also indicates that the observation of a sustained vortex gyration at zero magnetic field, required for targeted applications, is only possible if an out-of-plane polarizer is used (as in this work by applying an out-of-plane field) or if the polarizer is non-uniform or dynamically excited [33] , [34] , [35] . The quantitative agreement between our results and theory will also allow us to define the best condition to improve the efficiency of the spin transfer and microwave power, both in terms of device structure (for example, tilted or out-of-plane polarizer) and materials parameters (lower resistance-area product and larger MR ratios). Sample preparation The magnetic stacks grown by sputtering in a CANON ANELVA chamber contain a SAF and a free layer of NiFe separated by a thin MgO-insulating barrier: PtMn 15 nm/CoFe 2.5 nm/Ru 0.85 nm/CoFeB 3 nm/MgO 1.075 nm/NiFe 15 nm/Ru 10 nm. Details of the growth and fabrication process have been presented elsewhere [36] . The resistance-area product is 1.3 Ω μm 2 for the parallel magnetization configuration. At room temperature, the TMR ratio is 14% under a bias current I dc of 1.6 mA. The topology of the top NiFe layer has been investigated by means of atomic force microscopy (see Fig. 6b ). We find that the surface roughness is mainly due to a spacial distribution of the thickness of the polycrystalline NiFe layer. Indeed, the surface of the underlying MgO layer was observed to be much smoother than the NiFe layer. Characterization of the magnetic configuration Before the investigation of transport and microwave properties, a specific study was conducted by high-resolution spin-scanning electron microscope images obtained at zero magnetic field to characterize the actual magnetic structures on arrays of unconnected circular MTJs with different diameters d (see Supplementary Fig. 1 ). For d =72 nm, the remanent magnetic state is a single-domain state for all nanodots. By increasing the diameter to d =125 nm, a few dots remain in the single-domain state, whereas for most of them, the direction of the magnetic moments gradually changes to in-plane, leading to a contrast varying between black and white. For larger diameters, the most favourable configuration is eventually a single vortex state, in particular, for the diameter of d =170 nm chosen for this study. Experimental procedure The microwave response associated with current-induced vortex dynamics is studied by applying the magnetic field H perp out-of-plane and sweeping the DC I dc from 0 to 3.2 mA. At each current value, microwave measurements up to 1.5 GHz are recorded on a spectrum analyser after a 32 dB amplification. The background noise, measured at zero DC, is subtracted from the power spectra. In our convention, a positive current is defined as electrons flowing from the NiFe magnetic layer to the SAF layer. Micromagnetic simulation For simulations, we use our finite-difference micromagnetic code SpinPM. The simulated NiFe disk has a diameter of 170 nm, with a thickness of 15 nm. The mesh cell size is set to 2×2×3.75 nm 3 . We considered the following magnetic parameters: α =0.01 for Gilbert damping, 4π M s NiFe =9.0 kOe for the magnetization of the NiFe layer and 4π M s SAF =10.3 kOe for the effective magnetization of the polarizer (extracted from the experimental TMR curves). Spin polarization has been set to P spin =0.53 (the optimum polarization to reproduce the experimental frequency versus the field curve of Fig. 2 ). How to cite this article: Dussaux, A. et al . Large microwave generation from current-driven magnetic vortex oscillators in magnetic tunnel junctions. Nat. Commun. 1:8 doi: 10.1038/ncomms1006 (2010).